Parallel evolution ofcoxgenes in H2S-tolerant fish as key adaptation to a toxic environment Populations that repeatedly adapt to the same environmental stressor offer a unique opportunity to study adaptation, especially if there are a priori predictions about the genetic basis underlying phenotypic evolution. Hydrogen sulphide (H 2 S) blocks the cytochrome-c oxidase complex (COX), predicting the evolution of decreased H 2 S susceptibility of the COX in three populations in the Poecilia mexicana complex that have colonized H 2 S-containing springs. Here, we demonstrate that decreased H 2 S susceptibility of COX evolved in parallel in two sulphide lineages, as evidenced by shared amino acid substitutions in cox1 and cox3 genes. One of the shared substitutions likely triggers conformational changes in COX1 blocking the access of H 2 S. In a third sulphide population, we detect no decreased H 2 S susceptibility of COX, suggesting that H 2 S resistance is achieved through another mechanism. Our study thus demonstrates that even closely related lineages follow both parallel and disparate molecular evolutionary paths to adaptation in response to the same selection pressure. The power of evolution is nowhere more impressively apparent than in species thriving in extreme environmental conditions that are deleterious to their closest relatives. Examples for such extreme habitats are hydrogen sulphide (H 2 S)-rich waters, because H 2 S is a potent inhibitor of aerobic respiration. Even at low concentrations dissolved H 2 S blocks the cytochrome-c oxidase complex (COX) in the mitochondrial respiratory chain [1] . Though reversible, H 2 S effectively stops the ATP-generating oxidative phosphorylation pathway and may be acutely lethal for most metazoans if concentrations exceed a certain threshold [1] . Nevertheless, tolerance to high environmental H 2 S concentrations is known from a few taxa, including some freshwater fish [2] . Several populations in the Poecilia mexicana species complex can obviously cope with environmental H 2 S concentrations averaging up to 190 μM, as they occur in volcanic springs and adjacent non-sulphidic waters in Southern Mexico. Reciprocal translocation experiments demonstrated that this H 2 S tolerance is due to evolutionary adaptation and not an inherent, inducible feature of the species: the sulphidic habitat is always lethal for individuals from non-sulphidic populations, but also transferring individuals from sulphide habitats to non-sulphidic habitats increases their mortality, sometimes drastically, thus effectively constraining gene flow even among proximate populations in different habitat types [3] , [4] . The molecular mechanism of acute H 2 S toxicity is mainly the non-competitive binding of its neutral form to the haem a 3 /Cu B of the binuclear centre within the COX1 subunit [1] . The COX1 subunit is—together with the two other subunits COX2 and COX3 of the protein’s catalytic core—encoded in the mitochondrial genome by the genes cox1 , cox2 and cox3 , respectively. While it has been proposed that COX ‘cannot be the primary locus of sulphide adaptation’ in animals [2] , we tested the hypothesis that reduced H 2 S susceptibility of the COX represents a key adaptation allowing for the colonization and exploitation of sulphide-rich habitats by P. mexicana . To infer the molecular basis and evolutionary processes causing the observed tolerance of several populations in the P. mexicana species complex, we sampled individuals from sulphidic and non-sulphidic habitats from three drainages, the Ríos Pichucalco (Pich), Puyacatengo (Puy) and Tacotalpa (Tac). These populations belonged to P. mexicana sensu stricto , except for two H 2 S-adapted populations in the Pichucalco drainage (Pich-S1 and Pich S-2), which were described as P. sulphuraria [5] . Here, we demonstrate that decreased H 2 S susceptibility of COX evolved in parallel in two sulphide lineages, as evidenced by shared amino acid substitutions in cox1 and cox3 genes. One of the shared substitutions likely triggers conformational changes in COX1 blocking the access of H 2 S. In a third sulphide population, we detect no decreased H 2 S susceptibility of COX, suggesting that H 2 S resistance is achieved through another mechanism. Our study thus demonstrates that even closely related lineages follow both parallel and disparate molecular evolutionary paths to adaptation in response to the same selection pressure. COX activity To address our hypothesis, we designed a COX activity assay. Because isolated vertebrate COX is inhibited by half at a concentration of about 0.2 μM [6] , we tested relative COX activity at H 2 S concentrations of 0.0, 0.1, 0.3 and 0.5 μM. This is much lower than measured ambient concentrations; however, the outer body wall (see Supplementary Fig. 1 ) and both the cell and mitochondrial membrane provide effective barriers for H 2 S diffusion despite its lipid solubility [1] . The relative COX activity of individuals from non-sulphidic populations dropped significantly at the highest H 2 S concentration tested (between 36% activity loss in Puy and 73% in Pich), while those from all but one of the sulphidic habitats (Pich-S1, Pich-S2 and Puy-S) remained virtually unchanged ( Fig. 1 ). In contrast, the COX from Tac-S individuals was as susceptible as those of non-sulphidic populations (46% activity loss, Fig. 1 ). 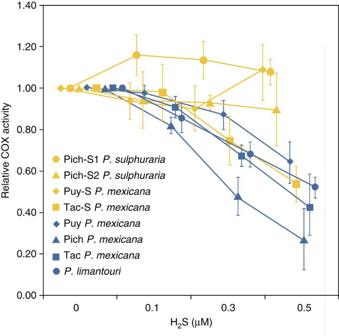Figure 1: COX activity changes differently when exposed to increasing H2S concentrations. Depicted is the mean (±s.d.n=8 except forn=6 andn=5) of relative COX activity of individuals from sulphidic (yellow symbols) and non-sulphidic (blue symbols) habitats measured at 0.0, 0.1, 0.3 and 0.5 μmol H2S. Figure 1: COX activity changes differently when exposed to increasing H 2 S concentrations. Depicted is the mean (±s.d. n =8 except for n =6 and n =5) of relative COX activity of individuals from sulphidic (yellow symbols) and non-sulphidic (blue symbols) habitats measured at 0.0, 0.1, 0.3 and 0.5 μmol H 2 S. Full size image Phylogenetic analysis of mitochondrial genomes We also tested whether non-susceptible COXs evolved independently in different lineages of sulphide spring populations and applied Bayesian phylogenetic analysis to nearly complete mitochondrial genomes of one individual per sampling site ( Fig. 2 ). In addition, one specimen of the species P. limantouri from Eastern Mexico, the presumed sister lineage to P. sulphuraria [3] , was included. The results indicated that the mitochondrial genomes of the P. mexicana lineages inhabiting sulphidic waters in Tac and Puy evolved independently from P. sulphuraria ( Fig. 1b , log Bayes factor unconstrained versus monophyly of sulphidic lineages >30). Applying a cytochrome b molecular clock rate estimated for a cave fish [7] indicated that the most recent common ancestor of all P. mexicana mitochondrial lineages is probably not older than 100 ka, while P. sulphuraria split between 200 and 500 ka from the P. limantouri -lineage ( Fig. 2 ). 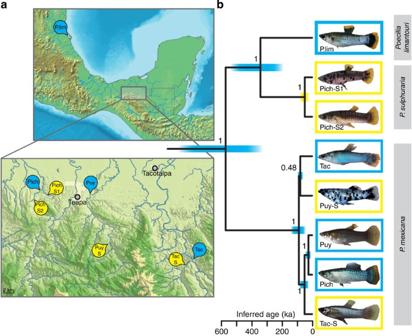Figure 2: Mitochondrial phylogeny of thePoecilia mexicanaspecies complex. (a) Map of Mexico, showing the sampling sites of the populations analysed. Symbols for populations from non-sulphidic sites are blue, those for sulphidic habitats yellow. (b) Bayesian molecular clock phylogeny of mitochondrial genomes from individuals from the eight study populations. Numbers above the branches indicate posterior probabilities. The tree was rooted with the mitochondrial genome ofXiphophorus maculatus(GenBank accession no. AP005982). Frames around pictures of representative individuals from the respective populations are coloured according to the habitat type. Shades beneath nodes indicate the 95% densities for the node age, their colour the parsimoniously reconstructed ancestral habitat (blue for clear water, yellow for sulphidic habitat). The analysis indicates that (i) the mitochondrial lineages in the sulphide habitats arose independently from each other out of ancestors from non-sulphidic water and (ii) the lineages withinP. mexicanaare not older than 100 ka, while theP. sulphurarialineage is between 200 and 500 ka old. Figure 2: Mitochondrial phylogeny of the Poecilia mexicana species complex. ( a ) Map of Mexico, showing the sampling sites of the populations analysed. Symbols for populations from non-sulphidic sites are blue, those for sulphidic habitats yellow. ( b ) Bayesian molecular clock phylogeny of mitochondrial genomes from individuals from the eight study populations. Numbers above the branches indicate posterior probabilities. The tree was rooted with the mitochondrial genome of Xiphophorus maculatus (GenBank accession no. AP005982). Frames around pictures of representative individuals from the respective populations are coloured according to the habitat type. Shades beneath nodes indicate the 95% densities for the node age, their colour the parsimoniously reconstructed ancestral habitat (blue for clear water, yellow for sulphidic habitat). The analysis indicates that (i) the mitochondrial lineages in the sulphide habitats arose independently from each other out of ancestors from non-sulphidic water and (ii) the lineages within P. mexicana are not older than 100 ka, while the P. sulphuraria lineage is between 200 and 500 ka old. Full size image Population genetic analyses The sulphidic lineages of P. mexicana in Tac and Puy appear to have evolved independently from each other as evidenced by nuclear markers (microsatellites, Supplementary Fig. 2a ). Population-level analysis of mitochondrial haplotype variation of 875 bp cox1 from 135 individuals revealed that the Tac-S population shares haplotypes with non-sulphidic populations, either as a result of on-going mitochondrial gene flow or shared ancestral polymorphisms ( Supplementary Fig. 2b ). In contrast, the Puy-S population was composed of a divergent, monophyletic mitochondrial lineage ( Supplementary Fig. 2b ). These haplotypes were exclusive to the Puy-S population and not found in any population from non-sulphidic habitats. Given our sampling scheme, the probability of detecting tolerant haplotypes in non-sulphidic populations is greater than 90% if the frequency of these haplotypes is at least 2%. Amino acid evolution Analysing the translated amino acid sequences of cox genes in a network approach revealed convergent amino acid substitutions in the cox1 and cox3 alleles shared by the non-susceptible COX types ( Fig. 3 ). In cox1 , an isoleucine–methionine (residue 75) and a valine–isoleucine (residue 435) substitution occurred independently in the Puy-S and Pich-S populations; the cox3 gene of the same populations shared an isoleucine–valine substitution at residue 61. A branch-specific test of positive selection indicated that both cox1 and cox3 had significantly increased ratios of non-synonymous to synonymous nucleotide substitutions ( ω ) along the branches to tolerant COX haplotypes ( Supplementary Fig. 3 ), indicating that at least some of the amino acid substitutions in these genes were driven by positive selection. In addition, a relative rate test indicated that amino acid evolution of COX1 and COX3 subunits in P. sulphuraria and the Puy-S lineage was significantly faster relative to their respective sister groups, while this was not the case for the Tac-S lineage ( Supplementary Table 1 ). 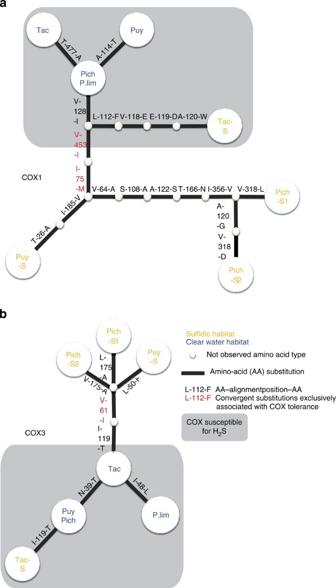Figure 3: Changes in amino acid compositions of COX subunits 1 and 3. Parsimonious amino acid network showing differences in amino acid compositions; each circle represents a particular amino acid composition of a COX subunit. The circles are connected by lines representing single amino acid substitutions. Large circles represent observed amino acid compositions, small circles inferred intermediates. Font colour indicates the habitat of origin for the respective lineage (blue non-sulphide habitat, yellow sulphidic habitat). Grey underlying shades signify subunits from H2S susceptible COX. Please note that this schematic is not a representation of the course of COX evolution. (a) Amino acid composition differences in COX1. Two amino acid substitutions at alignment positions 75 and 453 (in red) arose in parallel in the lineages with non-susceptible COX. (b) Amino acid composition differences in COX3. One amino acid substitution on alignment position 61 is common for all lineages with non-susceptible COX Figure 3: Changes in amino acid compositions of COX subunits 1 and 3. Parsimonious amino acid network showing differences in amino acid compositions; each circle represents a particular amino acid composition of a COX subunit. The circles are connected by lines representing single amino acid substitutions. Large circles represent observed amino acid compositions, small circles inferred intermediates. Font colour indicates the habitat of origin for the respective lineage (blue non-sulphide habitat, yellow sulphidic habitat). Grey underlying shades signify subunits from H 2 S susceptible COX. Please note that this schematic is not a representation of the course of COX evolution. ( a ) Amino acid composition differences in COX1. Two amino acid substitutions at alignment positions 75 and 453 (in red) arose in parallel in the lineages with non-susceptible COX. ( b ) Amino acid composition differences in COX3. One amino acid substitution on alignment position 61 is common for all lineages with non-susceptible COX Full size image Protein structure modelling To shed light on the molecular mechanism by which the observed amino acid changes may influence COX susceptibility, we modelled three dimensional protein structures. Our protein models indicate significant structural changes potentially relevant for the molecular function of COX1: particularly the isoleucine–methionine substitution at residue 75 in an alpha helix induces a hydrophobic interaction with a neighbouring alpha helix [8] , thereby changing the conformation of the two helices ( Fig. 4 ). 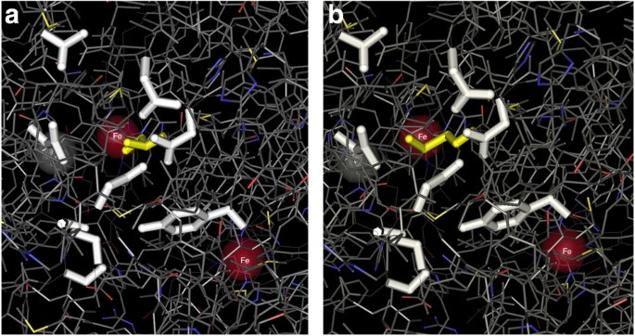Figure 4: Visualizations from structural protein modelling. Shown is the D-pathway channel in COX1. The conserved amino acid side chains lining the channel are highlighted in white, amino acid position 75 in yellow. In the background, the iron (red) and copper (grey) ions of the binuclear centre are depicted. (a) Protein structure as inferred from the translated amino acid sequence of a Pich individual, (b) same view for a Pich-S1 individual. The amino acid substitution at position 75 from isoleucine (a) to methionine (b) renders the channel narrower and thus, putatively less passable for H2S. Figure 4: Visualizations from structural protein modelling. Shown is the D-pathway channel in COX1. The conserved amino acid side chains lining the channel are highlighted in white, amino acid position 75 in yellow. In the background, the iron (red) and copper (grey) ions of the binuclear centre are depicted. ( a ) Protein structure as inferred from the translated amino acid sequence of a Pich individual, ( b ) same view for a Pich-S1 individual. The amino acid substitution at position 75 from isoleucine ( a ) to methionine ( b ) renders the channel narrower and thus, putatively less passable for H 2 S. Full size image As hypothesized, the COX activity assay revealed that this oxidative phosphorylation complex is at least in two cases involved in H 2 S tolerance of these fishes ( Fig. 1 ). Our results thus provide the first conclusive evidence of substantial differences in the sensitivity of COX to sulphide. Both P. sulphuraria populations (Pich-S1 and Pich-S2) and the Puy-S population of P. mexicana showed little or no decline of COX activity at concentrations that substantially inhibited the COX of fishes from non-sulphidic habitats. The unexpected susceptibility of COX from the independently evolved Tac-S population suggests the existence of a mechanism of H 2 S tolerance independent of COX (including its nuclear-encoded components) evolution. Detoxification mechanisms could indeed provide a complementary coping strategy in populations with a tolerant COX and an alternative strategy in the population with a susceptible COX. The gene encoding sulphide:quinone oxidoreductase, a conserved protein that catalyses the first step of enzymatic H 2 S oxidation in many metazoans [9] is consistently higher expressed in natural sulphide spring populations. Furthermore, common garden reared Tac-S individuals retain higher constitutive expression of this gene even in the absence of environmental H 2 S in the laboratory [10] . This indicates that adaptation to H 2 S may include mechanisms that reduce adverse effects of elevated exogenous concentrations (like a tolerant COX) and mechanisms that maintain low internal concentrations despite the constant influx of environmental H 2 S. Phylogenetic hypothesis testing showed that the non-susceptible P. sulphuraria and P. mexicana lineages arose independently and at different timescales ( Fig. 2 ). This rules out that the COX tolerance in P. mexicana observed in the Puy-S population is due to mitochondrial capture [11] via hybridization from P. sulphuraria or vice versa. If mutations in the mitochondrially encoded cox genes are indeed responsible for the observed COX tolerance, we would expect the Puy-S population to differ consistently in this regard from the other P. mexicana populations. Indeed, all Puy-S individuals screened possessed a divergent, monophyletic haplotype lineage that was not found in any other population. This suggests that (i) the tolerant COX lineages likely arose by de novo mutations and not from standing genetic variation [12] and (ii) mitochondrial gene flow among sulphide and non-sulphide populations is exceedingly rare in either direction. On the other hand, individuals from the Tac-S population shared haplotypes with most other non-sulphidic populations. This fits well with the observation that the COX of this population was equally susceptible as those of the non-sulphidic populations ( Fig. 2 ). Interestingly, the pattern of nuclear differentiation was exactly reversed in the Tac-S and Puy-S populations: the Tac-S population, sharing mitochondrial haplotypes with non-sulphidic populations, appeared completely isolated at nuclear loci, while there was substantial gene flow between the Puy-S population and the adjacent non-sulphidic population [3] . Rampant gene flow at selectively neutral microsatellite loci, but complete mitochondrial isolation among the adjacent Puy and Puy-S populations suggests that both mitochondrial lineages are selected against in the respective other habitat. Given that the mitochondrial lineages evolved independently, the identical amino acid substitutions in COX1 and COX3 ( Fig. 3 ) must have evolved in parallel. Such repeated trait changes in response to similar selective regimes are indicative of adaptive evolution [13] , a view that is substantiated by the significant test of positive molecular selection and the increased rate of amino acid evolution. Therefore, the respective amino acid substitutions (positions 75 and 453 in COX1 and 61 in COX3) are prime candidates for a key change in molecular function. While we could not infer a putative functional change for the latter two from protein modelling, the isoleucine–methionine substitution at position 75 in COX1 affected two helices that are part of the conserved D-pathway [8] . Protons (H + ) are pumped through this water-filled cavity towards the binuclear centre [14] , which likely also provides the access for H 2 S. We hypothesize that the predicted conformational change blocks the entrance to the D-pathway channel for the relatively large H 2 S molecules, but not for the considerably smaller H 2 O ( Fig. 4 ). We demonstrate that H 2 S-tolerant phenotypes in the P. mexicana species complex arose at least three times in parallel from ancestors living in non-sulphidic habitats. In two cases, we identified a parallel molecular basis with identical amino acid substitutions in two COX subunits, driven by natural selection as initially hypothesized. Against expectation [12] , this parallel evolution was highly unlikely to have drawn on standing genetic variation, but the necessary mutations arose independently (that is, de novo ). In one case, we could show that H 2 S tolerance is not due to COX evolution, but additional research is required to unravel its molecular basis. The present study is thus strengthening the conclusion derived from research on stickleback (reviewed in ref. 12 ) that the evolution of parallel phenotypes is often associated with a combination of identical mutations, different mutations in homologous genes, and the involvement of different genes. Sampling Adult fish were caught in sulphidic and non-sulphidic sites in all three drainages using seines ( Fig. 1 ; for sample sizes for the different analyses see the Supplementary Table 2 ). Fin clips for molecular genetic analyses were stored in 70% ethanol. Fish for the COX activity assay were placed in aerated, water-filled coolers and transported alive within 3 days upon capture to Oklahoma State University, where they were immediately decapitated, dissected livers stored in liquid nitrogen and shipped frozen to Frankfurt. Individuals for the COX activity from Tac and P. limantouri came from large, randomly outbred laboratory stocks maintained at the University of Frankfurt. COX activity assay Activity of cytochrome-c oxidase (EC 1.9.3.1) was measured for 5–8 wild-caught individuals from each population by a spectrophotometric method based on the oxidation of reduced cytochrome-c (ferrocytochrome-c) [15] . 1.0% (w/v) reduced cytochrome-c was prepared by dissolving 100 mg cytochrome-c (Sigma-Aldrich cat. no. C2506) in 8 ml 10 mM potassium phosphate buffer, pH 7.0, and addition of 4 mg L-ascorbic acid (Sigma-Aldrich cat. no. A7631). Excess ascorbic acid was then removed by dialyzing against 10 mM potassium phosphate buffer, pH 7.0 (Slide-A-Lyzer cassette, Pierce Chemicals), which resulted in a final volume of 10 ml. Aliquots of the solution—which is equivalent to 0.8 mM reduced cytochrome-c—were kept at −20 °C until use. Mitochondria were enriched from liver tissue by differential centrifugation [16] , [17] . Briefly, liver tissue was weighed and homogenized on ice in 1.5 ml microcentrifuge tubes with 10 volumes (10 μl mg −1 ) extraction buffer (20 mM Tris–HCl, pH 7.4, 200 mM sucrose, 130 mM NaCl) and a polypropylene pestle. After centrifugation at 1,500 g and 4 °C for 10 min the supernatant was collected and further centrifuged at 10,000 g and 4 °C for 12 min. The supernatant was discarded and the pellet comprising the mitochondria was resuspended in 1/10 of the volume extraction buffer that was used for homogenization. To break the mitochondria and to release COX, the tube was frozen in liquid nitrogen and rethawed three times. COX activity was measured in 1 ml reaction volume according to established methods based on the decrease in absorbance at 550 nm of ferrocytochrome-c caused by its oxidation to ferricytochrome-c by cytochrome-c oxidase [17] . Briefly, plastic cuvettes were filled with 915 μl 10 mM potassium phosphate buffer, pH 7.0, and 65 μl reduced cytochrome-c (53 μM final concentration in reaction). The cuvettes were kept at 25 °C before 20 μl of sample was added. Immediately after mixing thoroughly the decrease in the absorption at 550 nm was monitored for 10 min in a Hitachi U-2000 spectrophotometer. As a blank sample, 20 μl of a 100 mM potassium ferricyanide (Sigma-Aldrich cat. no. P8131) solution in 10 mM potassium phosphate buffer, pH 7.0, was added to the mixture instead of sample solution to completely oxidize the cytochrome-c. As a positive control for this assay, cytochrome-c oxidase from bovine heart (Sigma-Aldrich cat. no. C5499) dissolved to 0.02 mg ml −1 in 250 mM sucrose with 1% (v/v) Tween 80 was used. The difference in extinction coefficients between reduced and oxidized cytochrome-c is 21.84 at 550 nm [18] and one unit of COX activity is defined as the oxidization of 1.0 μM of ferrocytochrome-c per min at pH 7.0 at 25 °C, which was calculated using the following equation: where A × min −1 =decrease of A 550 nm per min in the reaction against the blank probe, dil=dilution factor of the sample or enzyme, 0.02=volume of the sample in ml. Protein content of the samples was assayed with 20 μl aliquots using the Bradford method [19] and comparisons with bovine serum albumin as standards. The COX activity was then determined in units per mg protein and the relative activity was plotted against H 2 S concentrations setting the value under control conditions as one. Measuring H 2 S influx through the body wall In our COX activity assay, we used H 2 S concentrations (0.0–0.5 μM) that were by orders of magnitude lower than ambient concentrations in sulphidic waters in Southern Mexico, where average (mean±s.d.) concentrations range between 23.7±18.2 and 190.4±119.7 μM [5] . This decision was made because the outer body wall and cellular and mitochondrial membranes are thought to be quite effective barriers to H 2 S influx [1] . To validate our approach and to demonstrate the efficacy of the outer body wall as a barrier to H 2 S influx, we killed N =6 laboratory-reared females from the susceptible Tac population (52.14±8.45 mm standard length, 3.37±1.36 g body weight) using an overdose of clove oil. A canal of app. 10 mm length was punctured into the caudal peduncle with a dissection needle to hold an H 2 S measuring device (Micro Sulphide Ion Electrode LIS-146AGSCM, Lazar Research Laboratories Inc., Los Angeles), approximately 2 mm beneath the outer body wall. The puncture opening was sealed with Vaseline. The probe was calibrated before all measurements using 10 −2 , 10 −3 , 10 −4 , 10 −5 and 10 −6 M Na 2 S-solutions, dissolved in antioxidant buffer (sodium salicylate, 391 mM, ascorbic acid, 92 mM, sodium hydroxide, 531 mM, dissolved in ddH 2 O, pH adjusted at 7.0). Test subjects were positioned head-first in a tube containing 20 ml of 40 mM Na 2 S solution (dissolved in antioxidant buffer, pH 7.0, at 22 °C). The experimental sulphide concentration was roughly 1,000 times higher than average ambient H 2 S concentrations in Mexican sulphide springs. Sequencing of mitochondrial genomes We used the DNA extractions of two fishes from the populations Pich and Tac-S to perform genomic shotgun sequencing on the Roche 454 next generation sequencing platform (a quarter plate for each fish) according to the manufacturer’s protocol. To identify reads of the mitochondrial genome, all 238,582 reads (average read length 354 bp) obtained for both fishes were blasted against the complete mitochondrial genome of another poeciliid fish, Xiphophorus maculatus (AP005982) with a cut-off value of e −10 . All identified mitochondrial reads were then assembled using the software Geneious (Geneious). From this consensus assembly, 18 overlapping primer pairs were developed with primer3 ( Supplementary Table 3 ). Direct traditional Sanger sequencing in both directions of the PCR products was then applied to one individual from eight populations. Thus, each base in the final genome versions was sequenced at least twice. The sequences were then assembled in Geneious. Annotation of protein coding genes, rDNAs, tDNAs and the d-loop was performed using the X. maculatus genome (AP005982) as reference and cross-checked with other fish mitochondrial genomes and the Ref-Seq database. Phylogenetic analyses We analysed all protein coding sequences, the partial 16S rRNA and the d-loop sequence of the nearly complete mitochondrial genomes with Bayesian methods implemented in the BEAST package [20] , using X. maculatus as outgroup. All partitions were analysed with an independent GTR+gamma+invariant sites model of molecular evolution, estimating all parameters during the analysis. We assumed that each partition evolved according to an independent uncorrelated relaxed clock model. We used a rate of 1.05 × 10 −8 mutations per year for the cytochrome b partition [7] to obtain a rough estimate of the approximate timescale of P. mexicana mtDNA evolution. All partition trees were coupled as appropriate for the non-recombining mtDNA. We ran the chain for 5 × 10 7 generations, sampling every 1,000th tree with a burn-in of 10% (after checking the level of convergence). The analysis was then repeated with identical parameters, but constraining the topology of the tree to monophyly of all sulphidic water lineages. The difference between both analyses was evaluated with log Bayes factors. We used the maximum clade credibility tree to infer the most likely ancestral habitat type (sulphidic or non-sulphidic) in Mesquite [21] under a maximum parsimony model of trait evolution. Population genetic analyses To infer a population genetic tree, we used a data set of 204 individuals of P. mexicana and P. sulphuraria published elsewhere [3] ; specimens were genotyped with 17 microsatellite markers (populations: Tac, Tac-S, Puy, Puy-S, Pich-S1: N =25 each; Pich: N =55; Pich-S2: N =24). We calculated Reynold’s pairwise distances using the software Arlequin v3.5.1.3 (ref. 22) [22] and inferred a neighbour joining tree from these distances using the programme Neighbour provided with the Phylip package [23] . For each of the 135 individuals from eight populations, we sequenced a 875 bp fragment of cox1 from both ends. Sequences were edited and aligned with Geneious (Geneious). We constructed a statistical parsimony network with the software TCS [24] . Amino acid type networks To identify shared and unique patterns of amino acid changes among varieties of COX proteins, we applied the principles of statistical parsimony haplotype network construction [25] to the amino acid sequences. Hence, each distinct amino acid composition (in analogy to a DNA sequence haplotype) was linked to the most similar type based on the minimum number of necessary amino acid substitution. Please note that this analysis does not represent an evolutionary reconstruction, as similar amino acid compositions can be reached via different evolutionary paths. Codon-based test of positive selection Tests on positive selection were performed by applying the codeml algorithm, implemented in the PAML programme package v. 4.4 (ref. 26) [26] to the alignments of all mitochondrial protein coding genes separately. Calculation of global ω values using the one ratio model was followed by calculation of branch-specific ω using the free ratio model. As the free ratio model is parameter rich and therefore prone to bias, only alignments with significantly better likelihood scores and with at least one non-synonymous substitution were used to infer positive selection. We used the inferred maximum clade credibility tree topology (see above) to calculate the branch-specific model. Relative rate test We tested for equality of substitution rates between pairs of COX amino acid sequences from the H 2 S-tolerant populations versus their respective sister taxon as inferred by phylogenetic analysis, using either P. limantouri or Pich as outgroup, with Tajima’s relative rate test [27] as implemented in MEGA5 (ref. 28) [28] . Three dimensional protein structure modelling The structures of COX1 and COX3 of the Pich and the Pich-S1 individual were modelled using SwissModel, a web-based tool for modelling the 3D atomic level structure of protein complexes [29] . The bovine COX crystal structure (Protein Data Bank ID IV54) was used as a template. The amino acid sequence of this template was about 89% similar for COX1 and about 80% similar for COX3. The models from SwissModel were visualized and interpreted in Cn3D [30] . Accession codes: All nucleotide sequences reproted in this study were deposited at GenBank (accession numbers KC992991 - KC992998 , KJ661407 - KJ661541 ). How to cite this article: Pfenninger, M. et al. Parallel evolution of cox genes in H 2 S-tolerant fish as key adaptation to a toxic environment. Nat. Commun. 5:3873 doi: 10.1038/ncomms4873 (2014).